Tetrahedrally coordinated carbonates in Earth’s lower mantle Carbonates are the main species that bring carbon deep into our planet through subduction. They are an important rock-forming mineral group, fundamentally distinct from silicates in the Earth’s crust in that carbon binds to three oxygen atoms, while silicon is bonded to four oxygens. Here we present experimental evidence that under the sufficiently high pressures and high temperatures existing in the lower mantle, ferromagnesian carbonates transform to a phase with tetrahedrally coordinated carbons. Above 80 GPa, in situ synchrotron infrared experiments show the unequivocal spectroscopic signature of the high-pressure phase of (Mg,Fe)CO 3 . Using ab-initio calculations, we assign the new infrared signature to C–O bands associated with tetrahedrally coordinated carbon with asymmetric C–O bonds. Tetrahedrally coordinated carbonates are expected to exhibit substantially different reactivity than low-pressure threefold coordinated carbonates, as well as different chemical properties in the liquid state. Hence, this may have significant implications for carbon reservoirs and fluxes, and the global geodynamic carbon cycle. Ferromagnesite ((Mg,Fe)CO 3 ) minerals are probable candidates for deep-Earth carbon storage and are expected to play a key role in the deep carbon cycle (for example, see refs 1 , 2 ). Therefore, the properties of ferromagnesite at lower mantle conditions have been the focus of many theoretical and experimental studies [2] , [3] , [4] , [5] , [6] , [7] , [8] . Results of high-pressure experiments have suggested that the rhombohedral structure of magnesite (MgCO 3 ) is stable up to 115 GPa at 2,000–3,000 K, and that it transforms to a new structure at higher pressures [2] . On the other hand, first-principles calculations predict that magnesite transforms into a phase containing CO 4 tetrahedral groups at lower pressure (~82 GPa) [5] . Boulard et al . [6] proposed that magnesite and ferromagnesite adopt the theoretically proposed structure above 80 GPa at 2,300 K, based on in situ X-ray diffraction (XRD) and ex situ spectroscopy analysis on recovered samples (electron energy loss spectroscopy and scanning transmission X-ray microscopy performed at the C–K edge). However, these observations have been controversial for two reasons: (1) only LeBail refinements were performed on the high-pressure, high-temperature XRD data and, hence, determination of the atomic positions within the unit cell was not possible; (2) spectroscopic analyses were performed ex situ on recovered samples after temperature quenching and decompression to ambient conditions, where transmission electron microscopic analyses showed amorphization of the sample indicating the high-pressure crystal structure was not preserved. Here we report the first unequivocal evidence of tetrahedrally coordinated carbon in high-pressure carbonates, obtained by a combined experimental and theoretical study. We perform in situ synchrotron infrared spectroscopic studies on ferromagnesite in diamond anvil cells (DAC) and identify a unique vibrational signature present only in the high-pressure phase. We perform ab initio calculations of the infrared spectra, which allow us to assign this vibrational signature to asymmetric, sp 3 -like C–O bonds. In situ infrared spectroscopy characterization Magnesite and siderite (FeCO 3 ) form a solid solution at ambient conditions and adopt the same structure at high pressure and temperature, except that on substitution of Mg by Fe, the volume of the unit cell decreases by about 7% (ref. 6 ) (V(MgCO 3 )=351.7 Å 3 at 85 GPa and 2,400±150 K and V(Mg 0.25 ;Fe 0.75 CO 3 )=328.9 Å 3 at 80 GPa and 300 K).We note that only the Fe-bearing phase is temperature quenchable [6] , an important requirement for infrared spectra measurements in the DAC. We thus chose a natural sample of ferromagnesite with a composition (Mg 0.25 Fe 0.75 )CO 3 , which was measured with an electron microprobe. Here we refer to the high-pressure structure of ferromagnesite as post magnesite. In situ infrared experiments were performed at the National Synchrotron Light Source on the high-pressure infrared beamline U2A. Two experiments were conducted: (1) infrared spectra were collected on compression and decompression of (Mg 0.25 Fe 0.75 )CO 3 between 0 and 54 GPa at ambient temperature. As the sample was not heated, (Mg 0.25 Fe 0.75 )CO 3 did not transform into the post-magnesite structure, but only experienced an isostructural electronic spin transition around 50 GPa [9] , [10] . (2) In a second set of experiments, powdered (Mg 0.25 Fe 0.75 )CO 3 was compressed up to 103 GPa and then transformed into the post-magnesite phase when laser heated at ~2,100 K. In situ XRD was used to monitor the transformation into the post-magnesite phase ( Supplementary Fig. 1 ). Infrared spectra were recorded at the highest pressure of 103 GPa and during decompression of the post-magnesite phase back to 0 GPa at room temperature. At low pressure, ferromagnesite is composed of repeating, alternating layers of (CO 3 ) 2− radicals (anions) and layers of divalent, positively charged cations (Fe 2+ and Mg 2+ ) ( Fig. 1a ). The mid-infrared spectral absorption features result primarily from fundamental internal vibrations of the C–O bonds in the carbonate radical: the out-of-plane bending ( ν 2 ), the asymmetric stretch ( ν 3 ) and in-plane bending ( ν 4 ) modes (for example see, ref. 11 ). At ambient conditions, we measured these three modes on the polycrystalline carbonate phase (symmetry group: R-3C) at 867, 1,460 and 739 cm −1 , respectively ( Fig. 2a ). Frequency of ν 3 was determined using a thinner sample ( cf . Supplementary Fig. 2 ). These frequencies are in good agreement with those reported by previous infrared studies on iron-bearing carbonates [3] , [11] , [12] . Additional modes resulting from the combination of the three fundamental ones are also present: a band at 1,811 cm −1 , which stems from the combination of ν 1 + ν 4 , and one at 2,512 cm −1 , which corresponds to the combination 2 ν 2 + ν 3 (ref. 13 ). Under compression at room temperature, no additional infrared bands were observed; rather, a shift to higher wave numbers was detected for all infrared bands, except for the transverse-optical (TO) component of the ν 2 band, which exhibited a slight negative pressure shift (−0.29 cm −1 GPa −1 ). Such a shift is in agreement with previous studies on iron-bearing carbonates [3] and has been interpreted as stemming from the increased strength of the divalent cation–oxygen bonds under compression. We observed no hysteresis on decompression of the untransformed carbonate. 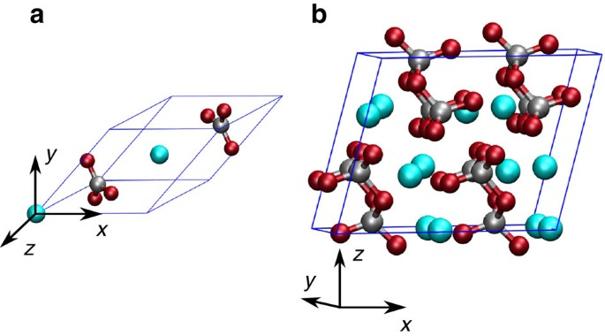Figure 1: Ball and stick representation of the two structures. Ferromagnesite at ambient conditions (a) and the post-magnesite phase above 80 GPa (b). Red, grey and blue spheres represent oxygen, carbon and cations (Fe or Mg) atoms, respectively. Figure 1: Ball and stick representation of the two structures. Ferromagnesite at ambient conditions ( a ) and the post-magnesite phase above 80 GPa ( b ). Red, grey and blue spheres represent oxygen, carbon and cations (Fe or Mg) atoms, respectively. 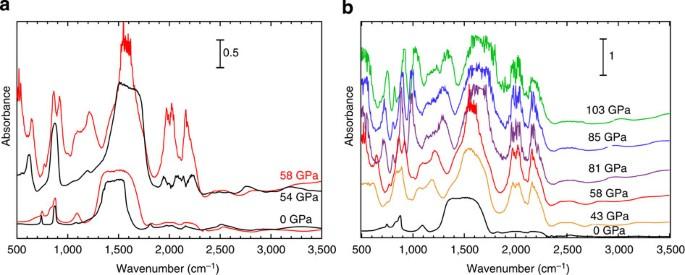Figure 2:In-situinfrared measurement at high pressure. (a) Experimental infrared spectra collected on compression of the ferromagnesite (black lines) at 0 and 54 GPa, and on decompression of the post-magnesite phase (red lines) at 58 and 0 GPa. The region between 1,900 and 2,300 cm−1is dominated by absorption from the diamond anvils. (b) Experimental infrared spectra collected on the decompression of the post-magnesite phase from 103 to 0 GPa. The scale bars give the absorbance scale for each panel. Full size image Figure 2: In-situ infrared measurement at high pressure. ( a ) Experimental infrared spectra collected on compression of the ferromagnesite (black lines) at 0 and 54 GPa, and on decompression of the post-magnesite phase (red lines) at 58 and 0 GPa. The region between 1,900 and 2,300 cm −1 is dominated by absorption from the diamond anvils. ( b ) Experimental infrared spectra collected on the decompression of the post-magnesite phase from 103 to 0 GPa. The scale bars give the absorbance scale for each panel. Full size image In the second set of experiments, several new infrared bands were observed after transformation into the post-magnesite phase by laser heating ( Fig. 2a ). At very high pressure (from 103 to 81 GPa), the most intense infrared bands appeared to be saturated, which made their positions difficult to determine precisely; however, our experiment showed that between 103 and 43 GPa these new infrared modes gradually shift to lower wavenumbers ( Fig. 2b ). At 0 GPa, the experimental spectrum does not correspond to a carbonate phase and displayed infrared modes at 746, 836, 872, 1,092, 1,480, 1,823, 2,349 and 2,530 cm −1 . We note that Boulard et al . [6] reported a redox reaction on laser heating of (Mg 0.25 Fe 0.75 )CO 3 , resulting in the formation of magnetite (Fe 3 O 4 ) together with the post-magnesite phase. However, the new infrared bands observed at ambient pressure after decompression cannot be assigned to magnetite [14] , [15] . First-principles calculations To interpret the infrared spectrum measured for the post-magnesite phase, we carried out first-principles calculations of the infrared spectra of MgCO 3 at low and high pressure, and we identified specific vibrational modes that are present only in the post-magnesite phase. Calculation were conducted for pure MgCO 3 instead of the solid solution, (Mg,Fe)CO 3 , for computational simplicity. We used density functional theory (DFT), a semi-local exchange-correlation (xc) functional [16] , plane-wave basis sets and pseudopotentials. We first calculated the infrared spectrum of magnesite (symmetry group: R-3C), the phase of MgCO 3 stable at ambient conditions (see Supplementary Fig. 3 ). We used a rhombohedral cell, with the lattice constant fixed at the experimental value of 5.675 Å and a cell angle of 48.2° (ref. 17 ; Supplementary Table 1 ). The computed frequencies of the TO component of the ν 2 , ν 3 and ν 4 modes are 825, 1,411 and 725 cm −1 , respectively. The theoretical frequencies computed for a single crystal are lower than the experimental ones by ~4% (refs 11 , 18 ). This discrepancy is probably due to the use of the semi-local xc functional Perdew–Burke–Ernzerhof [16] . By using the hybrid functional, B3LYP, Valenzano et al . [19] found a smaller error of ~0.5% for these three bands compared with the experimental results [11] , [18] . The infrared spectrum of the same magnesite structure computed at a pressure of 83 GPa, without allowing for any phase transition ( Supplementary Table 1 ), shows that the TO component of the ν 2 mode is weakly modified (we found a modest blue shift of 5 cm −1 ), the ν 4 mode (TO) is blue-shifted to 913 cm −1 and the ν 3 mode (TO) is blue-shifted to 1,647 cm −1 ( Supplementary Fig. 4 ). 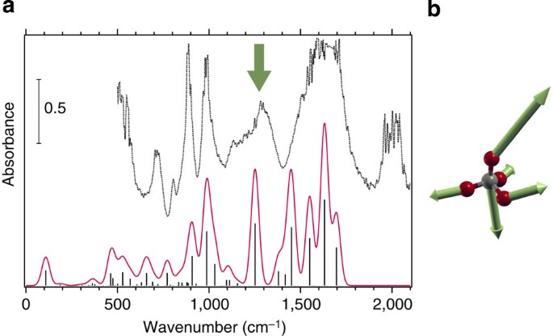Figure 3: Theoretical infrared results. (a) Calculated infrared intensities (black lines) and spectrum (solid red line) of the post-magnesite phase at 82 GPa. For comparison, the experimental spectrum collected at 81 GPa is shown as a dotted line. The scale bar gives the absorbance scale. (b) The vibrational mode at 1,252 cm−1(marked by the arrow ona) is identified as a unique signature of the high-pressure phase. Figure 3 shows the calculated infrared spectrum of the post-magnesite phase, compared with the experimental spectrum collected at ~81 GPa. We considered the structure of the post-magnesite (symmetry group: C2/m) previously measured for MgCO 3 at 82 GPa and high temperature (~2,300 K) by Boulard et al . [6] , with lattice constants a =8.39 Å, b =6.41 Å, c =6.82 Å and β =105.49° ( Supplementary Table 2 ). This structure is composed of tetrahedrally coordinated carbon atoms ( Fig. 1b ). In our computed spectrum, the phonon momentum is along the y axis (crystal direction: [010]) to take into account the longitudinal-optical (LO)–TO splitting (infrared spectra obtained by the TO component and the phonon momenta along the z and x directions are shown in Supplementary Fig. 5 ). We found three bands, at 659, 771 and 1,252 cm −1 , slightly red-shifted with respect to experiments (~715, 803 and 1,304 cm −1 ), again most probably because of the approximation introduced by the semi-local functional used in our calculations ( Supplementary Table 3 ). The two bands measured at 890 and 987 cm −1 were well reproduced by our calculations; we found 908 and 987 cm −1 , respectively. Overall, the theoretical and experimental spectra were in good agreement and, most importantly, they both exhibit a band at ~1,300 cm −1 , which is not present in magnesite at ambient conditions or in the infrared spectrum of the isotropically compressed magnesite phase ( Supplementary Fig. 4 ). The compressed magnesite does not exhibit any extra band between 1,000 and 1,400 cm −1 , providing strong evidence that the experimental and theoretical band at ~1,300 cm −1 signals the presence of a structural and bonding change. Figure 3: Theoretical infrared results. ( a ) Calculated infrared intensities (black lines) and spectrum (solid red line) of the post-magnesite phase at 82 GPa. For comparison, the experimental spectrum collected at 81 GPa is shown as a dotted line. The scale bar gives the absorbance scale. ( b ) The vibrational mode at 1,252 cm −1 (marked by the arrow on a ) is identified as a unique signature of the high-pressure phase. Full size image Our geometry optimization of the tetrahedrally coordinated post-magnesite phase showed that the CO 4 units, with nominal negative charge of four electrons, are asymmetric with both C and O atoms being sp 3 bonded, as shown in Fig. 4 , which reports hybrid orbitals (maximally localized Wannier functions [20] ) obtained from linear combinations of the eigenstates of the DFT Hamiltonian used in our calculations [21] . In the primitive cell of the high-pressure phase, carbon atoms have two symmetry non-equivalent positions, C1 and C2 (ref. 5 ). We found that for the CO 4 units consisting of the C1 atoms, the two longer C–O bonds are 1.427 and 1.375 Å, respectively, and the two shorter ones are 1.256 and 1.287 Å, respectively. For the other type of CO 4 units (C2 atoms), the two longer C–O bonds have the same length of 1.391 Å, while the two shorter ones are 1.285 and 1.276 Å, respectively. However, the bonding structure of these two units is similar and represented in both cases by the hybrid orbitals shown in Fig. 4 . The vibrational modes corresponding to the shorter C–O bonds are at frequencies higher than 1,400 cm −1 . At 81 GPa ( Figs 2b and 3 ), the band at 1,452 cm −1 originates from the stretching mode of the 1.287 Å C–O bonds and the one at 1,550 cm −1 from the stretching mode of the 1.285 and 1.276 Å C–O bonds. Finally, the modes at 1,631 and 1,696 cm −1 are assigned to the stretching modes of the 1.256 Å C–O bonds. We note that in the experimental spectra, the bands between 1,400 and 1,700 cm −1 are saturated and individual modes cannot be identified. The vibrational mode at 1,252 cm −1 originates from the stretching mode of the 1.375 and 1.391 Å C–O bonds, with the phonon momentum along the y axis ( Fig. 3b ). The TO component of this mode is expected at 1,155 cm −1 . The bands between 1,100 and 1,300 cm −1 may stem from the different LO and TO components of the 1,252 cm −1 stretching mode found in the experimental spectrum. As shown in Supplementary Fig. 5 , when the phonon momentum is along the x or z directions, the frequency of the stretching mode of the longer C–O bonds is lower than 1,252 cm −1 . The intensities of the LO and TO components in powder transmission spectra depend on the size and shape of the powder particles. There is an apparent band at 1,304 cm −1 in the experimental spectrum, suggesting that the thickness of many sample particles on the y direction may be much less than the wavelength of exciting radiation (7.7 μm in air) [22] . 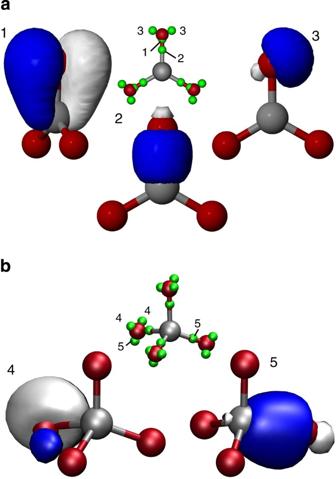Figure 4: Hybrid orbitals in C–O bonds. Threefold (a) and fourfold (b) coordinated carbon atoms in the magnesite and post-magnesite phases, respectively. Grey and red spheres represent C and O atoms, respectively. Green spheres represent the centres of the hybrid orbitals for the CO32−anion (a), with 24 valence electrons and 12 doubly occupied hybrids, and for the CO44−anion (b) with 32 valence electrons. The white and blue colours denote the positive and negative parts of the wave function, respectively. In magnesite both C and O aresp2bonded and three distinct orbitals were identified:σ-like orbitals localized on the C–O bonds (orbital 2),π-like bonds formed by the overlap ofpzorbitals on the O and C atoms (orbital 1) and lone pairs (orbitals 3) on the oxygen atoms; in post magnesite, both C and O aresp3bonded and two distinct orbitals were identified:σ-like orbitals localized on the C–O bonds (orbital 5) and lone-pair hybrids (orbitals 4) on the oxygen atoms. Hybrid orbitals were defined using maximally localized Wanier functions, built from linear combinations of single-particle electronic eigenstates (see Methods section). Figure 4: Hybrid orbitals in C–O bonds. Threefold ( a ) and fourfold ( b ) coordinated carbon atoms in the magnesite and post-magnesite phases, respectively. Grey and red spheres represent C and O atoms, respectively. Green spheres represent the centres of the hybrid orbitals for the CO 3 2− anion ( a ), with 24 valence electrons and 12 doubly occupied hybrids, and for the CO 4 4− anion ( b ) with 32 valence electrons. The white and blue colours denote the positive and negative parts of the wave function, respectively. In magnesite both C and O are sp 2 bonded and three distinct orbitals were identified: σ -like orbitals localized on the C–O bonds (orbital 2), π -like bonds formed by the overlap of p z orbitals on the O and C atoms (orbital 1) and lone pairs (orbitals 3) on the oxygen atoms; in post magnesite, both C and O are sp 3 bonded and two distinct orbitals were identified: σ -like orbitals localized on the C–O bonds (orbital 5) and lone-pair hybrids (orbitals 4) on the oxygen atoms. Hybrid orbitals were defined using maximally localized Wanier functions, built from linear combinations of single-particle electronic eigenstates (see Methods section). Full size image The modes detected between 1,100 and 1,300 cm −1 are at lower frequencies than the asymmetric stretching mode of the planar carbonate ion ν 3 measured at ambient conditions (1,401 cm −1 in this study). This is consistent with C–O bond lengths of 1.375~1.391 Å found in the CO 4 units, which are longer than that of the carbonate ion present in magnesite at ambient conditions (~1.30 Å). As expected, a longer bond length corresponds to a lower vibrational frequency. Such a trend was also found in magnesite by Grzechnik et al . [23] , who observed a shift of the ν 3 mode to lower frequency by ~114 cm −1 when decompressing the sample from 29 GPa to ambient conditions. Consistently, our calculation showed that when releasing the pressure of magnesite, from 58 to 0 GPa, the C–O bonds increase by 0.04 Å, and thus the TO component of the ν 3 mode redshifts by 194 cm −1 . In summary, we report the first in situ characterization of C–O bonds of the post-magnesite phase. We found that at high pressure, on transformation into the post-magnesite phase, the infrared spectrum of (Mg,Fe)CO 3 exhibits novel, unique features not present in the low-pressure spectrum, which we assigned to a fundamentally different bonding configurations of carbon. Carbon bonds transform from sp 2 (in the trigonal, doubly charged carbonate anions) to sp 3 hybridized configurations (in the tetrahedral tetra-charged carbonate anions), which we characterized using ab initio calculations within DFT. Hence, our study provides the identification of a mode at 1,304 cm −1 , which may be used as a fingerprint of tetrahedrally bonded carbon in high-pressure mineral phases. Carbon tetrahedrally bonded to oxygen has also been proposed to be present in high-pressure phase-V of CO 2 (refs 24 , 25 ). However, in this phase, tetrahedral CO 4 groups are symmetric with a C–O distance of 1.35 Å, similar to the longer C–O distances observed here. Measured infrared spectra showed the presence of a mode in the same frequency range at 1,126 cm −1 ; however, all modes were reported to involve simultaneous stretching and bending, unlike the pure stretching mode [24] identified here. The dramatic change we found in the carbon environment in ferromagnesite may have significant implications on carbon reservoirs and fluxes in the lower mantle and, therefore, on the deep carbon cycle. For example, the new bonding configuration, identified here in the high-pressure carbonate structure, is dramatically different from trigonal planar group in the ambient conditions structure. This will probably influence its chemical and physical properties such as its reactivity. Moreover, one would expect dramatic changes in the behaviour of carbonate melts with increases in coordination of carbon, owing to the ability of CO 4 to form polymerizable networks while CO 3 trigonal groups can not [26] . At upper mantle conditions, carbonate melts differ from silicate melts. They exhibit ultra-low viscosity potentially resulting in high mobilities [27] . Preliminary theoretical studies predict that carbonate melt viscosity increases at high pressures [28] , which would inhibit mobility of carbonate melts in the lower mantle and might lead to the presence of deep carbon reservoirs. In situ high-pressure infrared spectroscopy The infrared absorbance was measured in the 500–4,000 cm −1 range through a symmetric Mao-type DAC mounted with type-IIa diamond anvils. Measurements were conducted with a Bruker Vertex 80/v spectrometer at the side station of the high-pressure infrared beamline U2A of the National Synchrotron Light Source. The spectral resolution was 4 cm −1 and the beam size under the microscope was ~20 × 20 μm. Absorption infrared spectra were obtained after normalization against a background spectrum collected on an area with KBr pressure medium only (set 1) at each pressure or in the empty DAC (set 2) at ambient pressure. A natural sample of (Mg 0.25 Fe 0.75 )CO 3 siderite, provided by the mineralogical collection of University of Pierre et Marie Curie, was used in this experiment. For both sets of experiments, powdered (Mg 0.25 Fe 0.75 )CO 3 was loaded together with a ruby ball and the pressure was determined before and after infrared absorbance data collection from the shift of the ruby fluorescence line [29] . In the first set of experiments, KBr was added as a pressure-transmitting medium in a DAC with 400 μm culets. One run was performed with a sufficiently thin sample, to obtain good quality of the high-intensity band ν 3 , and a second run with a thicker sample, to get good data quality of the lower-intensity bands. In the second set of experiments, the sample was loaded without pressure medium in a DAC with 70 μm culets and compressed up to 103 GPa. The sample was then transformed into the post-magnesite phase by laser heating at ~2,100 K at HPCAT, Argonne National Laboratory. We used in-situ XRD to monitor the transformation into the post-magnesite phase. DFT calculations DFT calculations were performed with the Quantum ESPRESSO package [30] and maximally localized Wannier functions were computed with the Qbox code (v.1.56.2, http://eslab.ucdavis.edu/software/qbox/ ) [31] and the algorithm of reference [21] . We used the Perdew–Burke–Ernzerhof xc functional [16] , plane-wave basis sets and ultrasoft pseudopotentials [32] . We used a kinetic energy cutoff of 40 Ry for wavefunctions and 360 Ry for charge densities. Our structural optimizations were performed by fully relaxing all atomic coordinates within the primitive cell until the force on each atom was smaller than 10 −4 Ry Bohr −1 . We used 3 × 3 × 3 k -point mesh for the primitive cell of magnesite and 2 × 2 × 2 k -point mesh for the post-magnesite phase. We used the unit cell and atomic positions of the postmagnesite reported in Boulard et al . [6] in which the space group is P21/c after transferring the atomic positions from C2/m as reported in Oganov et al . [5] to P21/c. In the DFT calculations, the point group 2/ m was used. We carried out phonon calculations using density functional perturbation theory [33] to obtain the infrared spectra. The intensity of the m th infrared mode is defined as [34] : where α and β are Cartesian components, is the Born effective charge tensor of the s th atom and e m ( s , β ) is the normal mode eigenvector [34] . The calculated intensities were broadened by a Gaussian function with the full width of 50 cm −1 at half maximum. How to cite this article: Boulard, E. et al . Tetrahedrally coordinated carbonates in Earth’s lower mantle. Nat. Commun. 6:6311 doi: 10.1038/ncomms7311 (2015).